Twinned growth behaviour of two-dimensional materials Twinned growth behaviour in the rapidly emerging area of two-dimensional nanomaterials still remains unexplored although it could be exploited to fabricate heterostructure and superlattice materials. Here we demonstrate how one can utilize the twinned growth relationship between two two-dimensional materials to construct vertically stacked heterostructures. As a demonstration, we achieve 100% overlap of the two transition metal dichalcogenide layers constituting a ReS 2 /WS 2 vertical heterostructure. Moreover, the crystal size of the stacked structure is an order of magnitude larger than previous reports. Such twinned transition metal dichalcogenides vertical heterostructures exhibit great potential for use in optical, electronic and catalytic applications. The simplicity of the twinned growth can be utilized to expand the fabrication of other heterostructures or two-dimensional material superlattice and this strategy can be considered as an enabling technology for research in the emerging field of two-dimensional van der Waals heterostructures. The rational stacking of two different transition metal dichalcogenides (TMDCs, two-dimensional atomic crystalline materials with tunable electronic structure [1] , [2] , [3] , [4] , [5] and great potential in optoelectronic devices [6] , [7] , [8] , [9] , [10] ), has drawn significant attention as it endows TMDCs with great opportunities to expand their pristine properties [11] , [12] , [13] , [14] , [15] and broaden their applications [16] , [17] , [18] , [19] , [20] . Initially, vertically stacked heterostructures comprising multi-layered TMDCs were obtained by sequential mechanical exfoliation. These studies triggered subsequent studies focused on the top-down creation of TMDCs heterostructures with varied chemical composition, interlayer spacing, and angular alignment [11] . However, due to the limited size and randomly generated locations of the exfoliated TMDCs flakes, this stacking procedure is neither controllable nor scalable. Later, Ajayan et al . presented an approach for the chemical vapour deposition (CVD) synthesis of stacked WS 2 /MoS 2 heterostructures, which showed the potential for larger scale production [21] . However, due to the random nucleation process and poor control over the growth rate, it is extremely difficult to significantly increase the stacking area or to precisely control the growth behaviour of vertically stacked TMDCs heterostructures. Thus far, the stacking of two TMDCs constituents in a strictly controlled manner (especially in terms of control over the overlap percentage) has yet to be achieved, even though this is highly desirable. Herein, we demonstrate the twinned growth of two 2D (two-dimensional) nanomaterials, namely ReS 2 and WS 2 . We achieve 100% overlap for each of the stacked TMDCs structures, with crystal sizes of the heterostructures one order of magnitude larger than previous reports [12] , [13] , [14] , [16] , [18] , [20] , [21] , [22] , [23] , [24] , [25] , [26] . For the twinned growth of ReS 2 /WS 2 vertical heterostructures, Au is chosen as the substrate and W–Re alloy foil is used as the Re and W sources, which lower the barrier energies for this special twinned growth process. We believe that the developed approach will promote and accelerate ongoing research efforts of 2D crystalline van der Waals heterostructures. 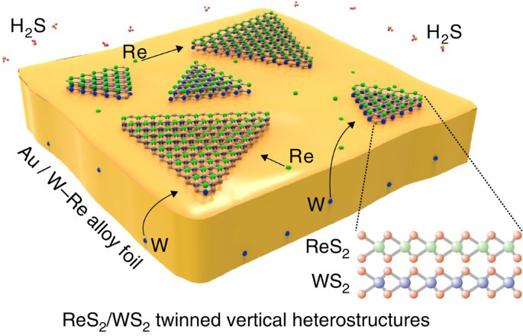Figure 1: Schematic for the twinned growth of ReS2/WS2. For the growth of ReS2/WS2twinned vertical heterostructures, Au is chosen as the growth substrate and W–Re alloy foil serves as the support substrate. This twinned growth process starts upon the introduction of H2S. The morphology and spectral characterization of ReS 2 /WS 2 Figure 1 schematically shows the strategy for the twinned growth of ReS 2 and WS 2 towards vertically stacked heterostructures. From scanning electron microscopy (SEM) images (for example, Fig. 2a ) taken from the Au surface after the CVD reaction, one can observe large-area uniformity and a high yield of triangular vertically stacked ReS 2 /WS 2 crystals. One can also see that the domain size of the smaller stacked ReS 2 /WS 2 structures is typically >10 μm, while the bigger crystal reaches a large size of 600 μm 2 ( Fig. 2a ). This is about 1 order of magnitude larger than other reports of vertically stacked TMDCs heterostructures synthesized by traditional CVD technique or by a sequential exfoliation process ( Fig. 2b ). Moreover, from Fig. 2b , we can also conclude that a 100% overlap of two TMDCs is obtained, and this is also much higher than previously reported findings. To further characterize the structure of the twinned ReS 2 /WS 2 crystals, the samples were transferred onto 300 nm Si/SiO 2 substrates. After transfer, typical optical image of the triangular crystal is shown as Fig. 2c , which reveals that the stacked ReS 2 /WS 2 structure exhibits a uniform light-purple triangle consistent with a high uniformity in agreement with the SEM data (representative image can be seen in Fig. 2a ). In addition, atomic force microscope images of the transferred crystals show a uniform height of ∼ 1.6 nm over the entire structure ( Supplementary Fig. 1 ), which confirms the bilayered, 100% overlapped structure and twinned growth nature of the ReS 2 /WS 2 heterostructures. Figure 1: Schematic for the twinned growth of ReS 2 /WS 2 . For the growth of ReS 2 /WS 2 twinned vertical heterostructures, Au is chosen as the growth substrate and W–Re alloy foil serves as the support substrate. 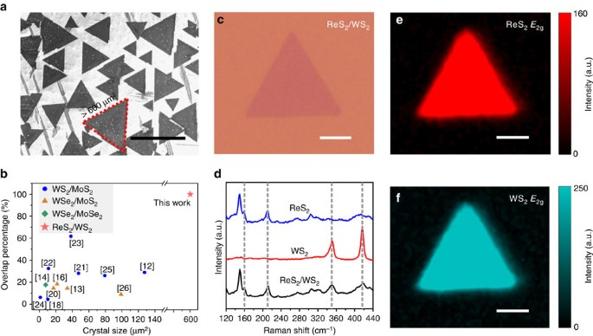Figure 2: Characterizations of ReS2/WS2twinned vertical heterostructures. (a) SEM image of the triangular ReS2/WS2vertical crystalline heterostructures over Au. A ReS2/WS2crystal with grain size up to 600 μm2is indicated. (b) Crystal size plotted as a function of overlap percentage of TMDCs heterostacks obtained in this work and those reported in other literature. (c) Optical image of a ReS2/WS2twinned vertical heterostructure crystal after transfer onto a Si/SiO2substrate. (d) Comparison of the Raman spectra of ReS2, WS2, and ReS2/WS2, in which four distinct peaks are observed from the twinned ReS2/WS2crystal (e,f) Raman mappings of peak intensity at 160.5 and 351.3 cm−1respectively, corresponding to theE2gmode of ReS2and WS2respectively. Scale bar, 40 μm (a); 5 μm (c,e,f). This twinned growth process starts upon the introduction of H 2 S. Full size image Figure 2: Characterizations of ReS 2 /WS 2 twinned vertical heterostructures. ( a ) SEM image of the triangular ReS 2 /WS 2 vertical crystalline heterostructures over Au. A ReS 2 /WS 2 crystal with grain size up to 600 μm 2 is indicated. ( b ) Crystal size plotted as a function of overlap percentage of TMDCs heterostacks obtained in this work and those reported in other literature. ( c ) Optical image of a ReS 2 /WS 2 twinned vertical heterostructure crystal after transfer onto a Si/SiO 2 substrate. ( d ) Comparison of the Raman spectra of ReS 2 , WS 2 , and ReS 2 /WS 2 , in which four distinct peaks are observed from the twinned ReS 2 /WS 2 crystal ( e , f ) Raman mappings of peak intensity at 160.5 and 351.3 cm −1 respectively, corresponding to the E 2g mode of ReS 2 and WS 2 respectively. Scale bar, 40 μm ( a ); 5 μm ( c , e , f ). Full size image Figure 2d shows the comparison between the Raman spectra of pure ReS 2 , pure WS 2 and the twinned ReS 2 /WS 2 heterostructure. Within the Raman spectrum of heterostructure, one can observe peaks from both ReS 2 ( E 2g ≈160.5 cm −1 and A 1g ≈211.3 cm −1 ) [27] and WS 2 ( E 2g ≈351.3 cm −1 and A 1g ≈417.8 cm −1 ) [28] . This shows that the structures are ReS 2 /WS 2 vertically stacked heterostructures and not an alloyed Re x W 1 −x S 2 crystal, since the Raman spectrum of a Re x W 1 −x S 2 alloy would show two main peaks with their positions between the E 2g and A 1g peaks of pure ReS 2 or WS 2 . To further confirm the 100% overlapped structure of the vertical heterostructures, Raman mapping was used. Typical examples are provided in Fig. 2e,f , in which Raman intensity maps using the ReS 2 E 2g mode at 160.5 cm −1 and the WS 2 E 2g mode at 351.3 cm −1 demonstrate a uniform response for both ReS 2 and WS 2 over the entire crystal. This rules out the possibility of alloying. In addition, Raman spectra were collected at fixed spatial positions at the center and corners of 11 randomly selected triangle ReS 2 /WS 2 crystals. Each verified the distinct signatures corresponding to ReS 2 and WS 2 ( Supplementary Fig. 2 ), so that the 100% overlapped structure and the large-scale twinned growth of the ReS 2 /WS 2 vertical heterostructures were further confirmed. Optoelectronic characterization of ReS 2 /WS 2 To explore the electronic structure of our ReS 2 /WS 2 twinned heterostructures, X-ray photoelectron spectroscopy (XPS) was implemented (see Fig. 3a and Supplementary Fig. 3 ). From the XPS data, the (Re and W):S atomic ratio is 1:2.0, indicating that the twinned ReS 2 /WS 2 is stoichiometric. As shown in Fig. 3b , comparison of the W 4f core level doublet from WS 2 and ReS 2 /WS 2 shows an up-shift of 300 meV, corresponding to a positive net charge on the WS 2 bottom layer [29] . Similarly, comparison of the Re 4f core level doublet from ReS 2 and ReS 2 /WS 2 shows a down-shift of 475 meV, corresponding to a negative net charge on the ReS 2 top layer [30] . Our results therefore indicate that the ReS 2 layer has a negative net charge, while the WS 2 layer has a positive net charge as a result of a contact potential. Hence the ReS 2 /WS 2 heterostructures serve as an atomically thin capacitor with a potential up to 775 meV, which originates from the work function difference induced charge transfer between the constituent ReS 2 and WS 2 layers and is twice that of previously reported TMDCs vertical heterostructures [20] . 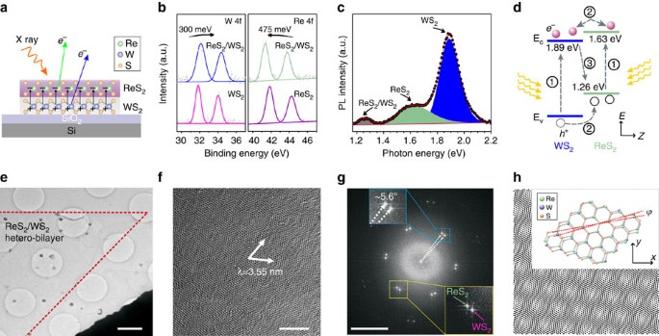Figure 3: Structure characterization of ReS2/WS2twinned vertical heterostructures. (a) Sketch of the X-ray photoelectron analyses of ReS2/WS2heterostack. (b) XPS core level shift analyses of ReS2/WS2heterostructures. (c) Photoluminescence spectrum of the ReS2/WS2heterostack, in which the three peaks are attributed to the exciton relaxations within ReS2(green), WS2(blue) and between ReS2/WS2layers (grey). (d) Band diagram of ReS2/WS2heterostructures under photo excitation, depicting (1) absorption and exciton generation in WS2and ReS2, (2) relaxation of excitons at the ReS2/WS2interface driven by the band offset, and (3) radiative recombination of spatially indirect excitons. (e) Low-magnification TEM image of the ReS2/WS2twinned vertical heterostructures, where a triangle crystal of ReS2/WS2hetero-bilayer is marked. (f) High-resolution TEM image of ReS2/WS2vertical heterostructures showing the resulting Moiré pattern. (g) Fast Fourier transform (FFT) of the heterostructures inf. The inset shows the two patterns of ReS2(green) and WS2(purple) with a rotation angle to be about 5.6°. (h) Tentative orientation model of rotating the upper ReS2by an angle of 5.6° with respect to the ground WS2. Insert is the atomistic illustration of the heterostructure of ReS2/WS2with their respective lattice constants and a misalignment angleϕ. Scale bar, 1 μm (e); 4 nm (f); 4 nm−1(g). Figure 3: Structure characterization of ReS 2 /WS 2 twinned vertical heterostructures. ( a ) Sketch of the X-ray photoelectron analyses of ReS 2 /WS 2 heterostack. ( b ) XPS core level shift analyses of ReS 2 /WS 2 heterostructures. ( c ) Photoluminescence spectrum of the ReS 2 /WS 2 heterostack, in which the three peaks are attributed to the exciton relaxations within ReS 2 (green), WS 2 (blue) and between ReS 2 /WS 2 layers (grey). ( d ) Band diagram of ReS 2 /WS 2 heterostructures under photo excitation, depicting (1) absorption and exciton generation in WS 2 and ReS 2 , (2) relaxation of excitons at the ReS 2 /WS 2 interface driven by the band offset, and (3) radiative recombination of spatially indirect excitons. ( e ) Low-magnification TEM image of the ReS 2 /WS 2 twinned vertical heterostructures, where a triangle crystal of ReS 2 /WS 2 hetero-bilayer is marked. ( f ) High-resolution TEM image of ReS 2 /WS 2 vertical heterostructures showing the resulting Moiré pattern. ( g ) Fast Fourier transform (FFT) of the heterostructures in f . The inset shows the two patterns of ReS 2 (green) and WS 2 (purple) with a rotation angle to be about 5.6°. ( h ) Tentative orientation model of rotating the upper ReS 2 by an angle of 5.6° with respect to the ground WS 2 . Insert is the atomistic illustration of the heterostructure of ReS 2 /WS 2 with their respective lattice constants and a misalignment angle ϕ . Scale bar, 1 μm ( e ); 4 nm ( f ); 4 nm −1 ( g ). Full size image Photoluminescence (PL) spectrometry was used to investigate the interaction between ReS 2 /WS 2 heterostack layers. As shown in Fig. 3c , three prominent peaks are observed at exciton transition energies of 1.89, 1.63 and 1.26 eV, corresponding to wavelengths of 657, 759 and 987 nm, respectively. The two strong exciton peaks at 1.63 eV (759 nm) and 1.89 eV (657 nm) are consistent with the PL intensities for ReS 2 and WS 2 , and are in good agreement with previous works [29] , [30] . The weak peak at 1.26 eV (987 nm) can be attributed to an indirect exciton transition between the ReS 2 and WS 2 layers. This interlayer PL exciton transition is a type II band alignment, which highlights the twinned growth nature of the ReS 2 /WS 2 layers forming the heterostructure. Figure 3d shows the band diagram for ReS 2 /WS 2 heterostructures under photo excitation. Owing to energy lost to the band offset, the PL exciton peak energy (1.26 eV) is lower than the excitonic band gaps for either of the TMDCs constituents (1.63 eV for ReS 2 or 1.89 eV for WS 2 ). Moreover, the strong luminescence signal at energies corresponding to the excitonic band gaps of ReS 2 (1.63 eV) and WS 2 (1.89 eV) suggests that a minority of the photoexcited carriers are relaxed at the interface leading to a low luminescence signal from the spatially indirect recombination process. Although the intensity of the indirect excitonic peak is weak, it is still an indication that the interface of the twinned ReS 2 /WS 2 is clean and contamination-free, which confirms the advantages of our strategy for the fabrication of high-quality TMDCs heterostructures. High-resolution characterization of ReS 2 /WS 2 To further reveal the crystalline structure and the stack orientation of the twinned ReS 2 /WS 2 heterostructures, high-resolution transmission electron microscopy (HRTEM) was utilized to characterize the samples after transferring them to a TEM grid or onto a Si/SiO 2 substrate. Low-magnification TEM image of a ReS 2 /WS 2 twinned vertical heterostructure is presented in Fig. 3e , in which the crystal edge is marked. The structural continuity within the ReS 2 /WS 2 domain suggests that our twinned vertical heterostructure is of high quality. Clear Moiré pattern, with periodicity measured to be about 3.55 nm, is observed in the high-resolution TEM image of the stacked structures as shown in Fig. 3f and the corresponding result of Fast Fourier transform is exhibited in Fig. 3g . Inspection of the Fast Fourier transform pattern reveals that in this particular sample the two hexagonal reciprocal lattices are rotated by ϕ =5.6° with respect to each other and there is negligible strain in the two constituent layers. Further simulation of the atomic structure by rotating the upper ReS 2 by the angle of ϕ with respect to the ground WS 2 layer ( Fig. 3h ) has shown similar Moiré pattern to that observed in Fig. 3f . To further confirm the stacked nature of the heterostructure, cross-section TEM samples were prepared by focused ion beam (FIB). The cross-sectional TEM images of ReS 2 /WS 2 heterostructure demonstrate the clean interface as well as the bilayer stacked structure of our twinned ReS 2 /WS 2 heterostacks ( Supplementary Fig. 4 ). To have a better understanding of the twinned growth behaviour between the ReS 2 and WS 2 layers on Au, we simulated the growth process of ReS 2 and WS 2 based on the density functional theory (DFT) calculations (as shown in Fig. 4 ). Before these first-principles calculations, however, X-ray diffraction investigations were conducted. The data confirmed that the Au substrate is crystalline ( Supplementary Fig. 5 ). When referenced with JCPDS data (JCPDS 04–0784), a clear match for Au (111) is obtained. Moreover, this was found for the entire surface, which confirms the single crystalline nature of our Au substrates. 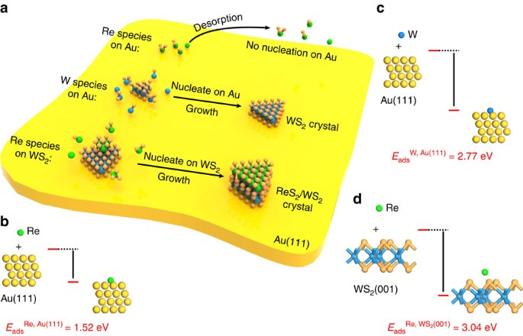Figure 4: Theoretical simulations confirming the twinned growth nature between ReS2and WS2. (a) Schematic illustrating the twinned growth of the ReS2/WS2heterostructures over Au(111). (b–d) Side views of the simulated surface adsorption of Re atoms (b) and W atoms (c) over Au(111) and Re atoms over WS2(001) facet (d). Figure 4: Theoretical simulations confirming the twinned growth nature between ReS 2 and WS 2 . ( a ) Schematic illustrating the twinned growth of the ReS 2 /WS 2 heterostructures over Au(111). ( b – d ) Side views of the simulated surface adsorption of Re atoms ( b ) and W atoms ( c ) over Au(111) and Re atoms over WS 2 (001) facet ( d ). Full size image Although the growth process of ReS 2 and WS 2 is complex, it can be simplified as follows [31] . The Re and W precursors are partially reduced by H 2 S gas to form a subsulfide species of ReS x and WS x ( x =1 ∼ 3), which are then further sulfurized into ReS 2 or WS 2 over the substrate (as shown in Fig. 4a ). To confirm the proposed mechanism, the adsorption energies for Re, W atoms over Au (111) and for Re atoms over WS 2 (001) were calculated using first-principles calculations within DFT. The adsorption results for these atoms on the different substrates are provided in Fig. 4b–d . From the data it is clear that the adsorption energies for W atoms over Au(111) and Re atoms on WS 2 (001) are very close to each other ( E ads W, Au(111) =2.77 eV, ). However, the adsorption energy for Re atoms over Au(111) ( E ads Re, Au(111) =1.52 eV) is far weaker. At the implemented high growth temperature of 900 °C this weak energy would easily be overcome, resulting in the facile desorption of Re species making the nucleation of ReS 2 highly unlikely. However, the strong adsorption energy (2.77 eV) is sufficiently accessible for WS 2 to nucleate and grow over Au (111). Once WS 2 forms on the substrate, the high adsorption energy of Re atom on WS 2 (001) would induce the subsequent adsorption, nucleation and growth of ReS 2 on the newly formed WS 2 surface. This beautifully highlights the twinned growth of ReS 2 /WS 2 crystals. To further confirm the twinned growth behaviour, different support substrates, namely, W foil, Re foil and W–Re alloy foil were investigated at a growth temperature of 900 °C. 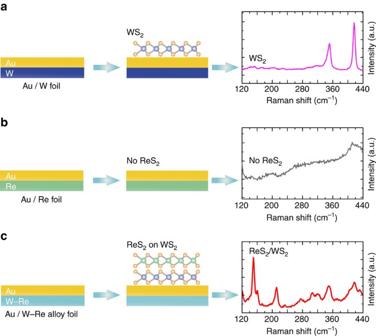Figure 5: Scheme and Raman data illustrating the twinned growth nature between ReS2and WS2. (a–c) Growth schematics and Raman spectra collected on Au while using W foil (a), Re foil (b) and W–Re alloy foil (c) as the support substrate. Figure 5 shows the scheme for the different support substrates and corresponding growth results. When W foil is used, WS 2 can easily form on the surface of Au(111) (see Fig. 5a and Supplementary Fig. 6 ), confirming the high adsorption energy of W atoms on Au(111). This allows the nucleation and growth of WS 2 on Au(111) at 900 °C. However, when Re foil is used as the support substrate, no ReS 2 Raman response is found on the Au(111) surface (as shown in Fig. 5b ). This indicates that ReS 2 is not obtained at 900 °C due to the facile desorption of Re atoms from Au(111) because of their low adsorption energy. However, when the W–Re alloy was used as the support substrate, four distinct peaks arising from the E 2g , A 1g modes of both ReS 2 and WS 2 are observed ( Fig. 5c ). This tells us that stacked ReS 2 /WS 2 heterostructures have formed and this is attributed to the preferential growth of WS 2 on Au and then the subsequent growth of ReS 2 on WS 2 (001) as discussed above. The data confirms that Re atoms are adsorbed on the WS 2 (001) surface enabling nucleation and growth of ReS 2 . In addition, it should be noted that the reaction temperature of 900 °C is very crucial for the dominance of the twinned growth behaviour in the process ( Supplementary Fig. 7 ). Figure 5: Scheme and Raman data illustrating the twinned growth nature between ReS 2 and WS 2 . ( a – c ) Growth schematics and Raman spectra collected on Au while using W foil ( a ), Re foil ( b ) and W–Re alloy foil ( c ) as the support substrate. Full size image Finally, we demonstrate the hydrogen evolution reaction activity for our ReS 2 /WS 2 twinned vertically stacked heterostructures ( Supplementary Fig. 8 ). The data show that our twinned heterostructures exhibit superior hydrogen evolution reaction activity as compared to pure WS 2 and own great potential as a catalytic material. Besides, our ReS 2 /WS 2 twinned vertical heterostructures also show better transfer performance than individual ReS 2 ( Supplementary Fig. 9 ). Furthermore, the strategy developed here is versatile as a general method for fabricating other TMDCs heterostructures. For example, MoS 2 /WS 2 vertical heterostructures could be fabricated using Mo-W alloy foils in place of the W–Re alloy foils during the growth process ( Supplementary Fig. 10 ). In summary, the use of a W–Re alloy foil as a supply source of Re and W atoms, along with the difference in the adsorption energies of Re and W atoms on Au(111) surfaces allows us to demonstrate the possibility of twinned growth between 2D nanomaterials. Importantly, the presented strategy is not limited to ReS 2 and WS 2 , which also allows the fabrication of other TMDCs vertical heterostructures such as MoS 2 /WS 2 . Besides, the strategy can be extended to any 2D material whose precursor possesses an appropriate adsorption energy at the required surface. A key factor is the correct choice of the reaction temperature to enable the selective growth of one nanomaterial over another. This type of 2D twinned vertically stacked heterostructures has a 100% overlap and their crystal sizes are one order of magnitude larger than previous reports. The simplicity of the process may be expanded to construct other vertically stacked or in-plane 2D heterostructures, thus, advancing research in the emerging field of 2D van der Waals heterostructures as well as the fundamental understanding of the nucleation and growth of TMDCs. The growth of ReS 2 /WS 2 twinned vertical heterostructures To achieve the one-step growth of ReS 2 /WS 2 twinned vertically stacked heterostructures, we utilized a re-solidified Au substrate in which Re and W atoms had been dissolved in. To prepare the special substrate, a piece of Au wire was placed on W–Re alloy foil. Under the protection of an Ar/H 2 atmosphere, the Au spread evenly over the entire foil by annealing at 1,100 °C for ∼ 10 min which also allows Re and W atoms diffuse into the Au lattice. After that, the temperature was decreased to 900 °C for the CVD growth reaction. The simultaneous growth of ReS 2 /WS 2 layers forming a vertically stacked heterostructure starts upon the introduction of H 2 S into the system for 10 min. This simple, scalable synthesis process is a direct CVD growth approach with no intermediate transfer steps. Characterization Scanning electron microscope images were taken by Zeiss Sigma. Optical images were taken with an optical microscope (Olympus DX51). Raman spectroscopy and photoluminescence with an excitation wavelength of 532 nm were carried out using a Renishaw inVia. The atomic force microscope images were collected on an NT-MDT Ntegra Spectra. The ReS 2 /WS 2 was transferred onto the 300 nm SiO 2 /Si for such measurements. X-ray photoelectron spectroscopy was performed on a Thermo Scientific, ESCALAB 250Xi. The measuring spot size was 500 μm and the binding energies were calibrated by referencing the C 1 s peak (284.8 eV). The TEM images were taken with an aberration corrected, high-resolution TEM (AC-HRTEM, FEI Titan [3] ) operating at 80 kV. X-ray diffraction measurements were performed using a Rigaku MiniFlex600 with Cu–Ka radiation over the range of 2 θ =10 ∼ 80°. DFT calculations The spin polarized density functional theory calculations were performed using the DMol3 (ref. 32 ) module in the Materials Studio software (Bio Accelrys). Exchange-correlation functional was based on Perdew-Burke-Ernzerh (PBE) within the generalized gradient approximation. The core electrons were treated with DFT semi-core pseudopotentials. The optimized lattice constant of Au is 4.180 Å, in good agreement with the experimental value of 4.078 Å. The Au(111) facet was modelled by an unreconstructed 4 × 4 surface slab, which contains four atomic layers with a vacuum region of ∼ 20 Å. The self-consistent-field (SCF) convergence criterion was set to be <10 −5 Hartree and the force convergence was set to be lower than 0.002 Hartree per Å for all the optimizations of the adsorptions. In particular, for the optimization of the adsorption of Re atoms and W atoms on Au(111) facets, the bottom two layers of Au atoms were fixed at their bulk positions. A 5 × 5 × 1 k-point mesh was used to sample the Brillouin zone of the supercells. The adsorption energy of a X (X=Re or W) atom on the surfaces of M (M=Au(111) or WS 2 (001)) substrate is defined as E ads X, M =E(M)+E(X)−E(M−X). Data availability The data that support the findings of this study are available from the corresponding author upon request. How to cite this article: Zhang, T. et al . Twinned growth behaviour of two-dimensional materials. Nat. Commun. 7, 13911 doi: 10.1038/ncomms13911 (2016). Publisher's note: Springer Nature remains neutral with regard to jurisdictional claims in published maps and institutional affiliations.